Aurora B potentiates Mps1 activation to ensure rapid checkpoint establishment at the onset of mitosis The mitotic checkpoint prevents mitotic exit until all chromosomes are attached to spindle microtubules. Aurora B kinase indirectly invokes this checkpoint by destabilizing incorrect attachments; however, a more direct role remains controversial. In contrast, activity of the kinase Mps1 is indispensible for the mitotic checkpoint. Here we show that Aurora B and Hec1 are needed for efficient Mps1 recruitment to unattached kinetochores, allowing rapid Mps1 activation at the onset of mitosis. Live monitoring of cyclin B degradation reveals that this is essential to establish the mitotic checkpoint quickly at the start of mitosis. Delayed Mps1 activation and checkpoint establishment upon Aurora B inhibition or Hec1 depletion are rescued by tethering Mps1 to kinetochores, demonstrating that Mps1 recruitment is the primary role of Aurora B and Hec1 in mitotic checkpoint signalling. These data demonstrate a direct role for Aurora B in initiating the mitotic checkpoint rapidly at the onset of mitosis. The anaphase-promoting complex/cyclosome (APC/C) is the ubiquitin ligase responsible for degrading cyclin B and securin to allow sister chromatid separation and mitotic exit (reviewed in ref. 1 ). The APC/C remains inhibited until all chromosomes are attached to microtubules via their kinetochores, because unattached kinetochores catalyse production of an APC/C inhibitor termed the mitotic checkpoint complex ((refs 2 , 3 , 4 , 5 ) and reviewed in ref. 6 ). A key step in this catalysis is the conformational activation of the checkpoint protein Mad2 to a form known as C-Mad2 (reviewed in ref. 7 ), which is able to bind to the APC/C coactivator protein Cdc20 and ultimately cause efficient APC/C inhibition. The initial recruitment of Mad2 to kinetochores and its subsequent conversion to C-Mad2 rely on the kinase Mps1 (refs 8 , 9 , 10 , 11 ). Chromosomes with erroneous kinetochore–microtubule attachments can indirectly engage the mitotic checkpoint by virtue of unattached intermediates that are formed during the error-correction process [12] , [13] . Error correction is mediated by the chromosomal passenger complex that contains Aurora B as its executioner kinase (reviewed in ref. 14 ). Aurora B is thought to cause release of faulty attachments via phosphorylation of Hec1 and other components of the KMN network that form the core microtubule-binding site at the kinetochore, thereby reducing its microtubule-binding affinity [15] , [16] , [17] , [18] . It is currently unknown whether Aurora B has more direct roles in the mitotic checkpoint, as studies using different experimental systems reached conflicting conclusions [13] , [19] , [20] , [21] , [22] , [23] . We show here that Aurora B activity is critical to establish the checkpoint quickly following mitotic entry in mammalian cells. Aurora B enhances the recruitment of Mps1 to unattached kinetochores, which is needed to achieve rapid Mps1 activation at the onset of mitosis. This is the primary direct role for Aurora B in the mitotic checkpoint as recovering Mps1 recruitment to kinetochores rescues all checkpoint phenotypes associated with Aurora B inhibition in nocodazole-arrested cells. Aurora B therefore directly impacts on mitotic checkpoint function by ensuring timely Mps1 activation as soon as cells enter mitosis. Aurora B inhibition delays Mps1 activation during mitosis We, along with others, have recently implicated Aurora B as a factor involved in kinetochore binding of inactive Mps1 (refs 24 , 25 ). To examine whether this function of Aurora B could impact on the mitotic checkpoint, localization and activity of Mps1 were monitored following mitotic entry in the presence of Aurora B inhibitors. To exclude the indirect effects of Aurora B inhibition on the mitotic checkpoint, which arise from its ability to affect kinetochore–microtubule interactions, these and all further experiments were performed in the presence of the microtubule-depolymerizing drug nocodazole (unless stated otherwise). Mps1 strongly localized to kinetochores during prophase and early prometaphase [26] ('early prometaphase' cells had lightly condensed chromosomes that were scattered in the cytoplasm in contrast to 'late prometaphase' cells that had a highly condensed chromosome mass typical of nocodazole-arrested cells; Fig. 1a,b ). Aurora B inhibition using the small molecules Hesperadin or ZM447439 (hereafter referred to as Hesp or ZM in all figures) [22] , [23] reduced Mps1 kinetochore binding throughout mitosis ( Fig. 1a,b ). To examine if this reduction in kinetochore binding affected Mps1 activity, we assayed Mad2 localization to kinetochores, which requires kinase activity of Mps1 (refs 8 , 9 , 10 , 11 , 25 and 27 ). This therefore enabled quantification of Mps1 activity within single cells. As expected [26] , Mad2 recruitment was initiated in prophase and peaked in the early prometaphase cells ( Fig. 1a,b ). In contrast to the reduction in Mps1 kinetochore binding throughout mitosis, Mad2 levels were only significantly affected by Aurora B inhibition during the early stages ( Fig. 1a,b ). Similar effects on localization of Mps1 and Mad2 were observed after short interfering RNA (siRNA)-mediated knockdown of Aurora B ( Supplementary Fig. S1 ). To confirm that Mps1 activity at kinetochores was directly affected by Aurora B inhibition, we used an antibody against the activation loop phosphorylation site in Mps1 (pT676). Phosphorylation of this site is needed for full Mps1 activity and has been used previously as a marker for Mps1 activation [28] . 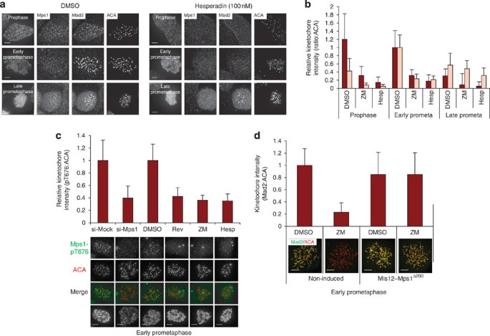Figure 1: Aurora B inhibition delays Mps1 activation at kinetochores. (a) HeLa cells treated with nocodazole containing DMSO or Hesperadin (100 nM) for 2 h and stained with the indicated antibodies. (b) Mean total kinetochore intensities (±s.d.) of Mps1 (dark red bars) or Mad2 (pink bars) relative to centromeres (ACA), treated as in (a) or with ZM447439 (2 μM). Data are from 20 cells from two experiments (Hesperadin treatment) or 40 cells from four experiments (DMSO and ZM447439 treatments). Ratios in early prometaphase are set to 1. (c) Example immunofluorescent images and quantification of kinetochore signal intensities of Mps1-pT676 over centromeres (ACA) in HeLa cells treated with nocodazole and indicated siRNAs or drugs. (d) Example immunofluorescent images and quantification of kinetochore signal intensities of Mad2 over centromeres (ACA) in U2OS cells, non-induced or induced to express LAP–Mis12–Mps1Δ200, and treated with nocodazole and indicate drugs. For panelscandd, ratio in si-Mock or DMSO-treated cells is set to 1 and mean data (±s.d.) are from 20 individual cells from two independent experiments. All images most closely resemble the mean values. All standard deviations represent the deviation in mean total kinetochore intensities between all individual cells analysed. Scale bars are 5 μm. For all experiments cells were treated with thymidine for 24 h, released into media containing nocodazole and indicated drugs for 10 h before fixation. siRNAs in panel c were transfected 16 h before the thymidine arrest. Figure 1c shows that kinetochore-localized pT676 was reduced during the early prometaphase following Mps1 knockdown or inhibition, validating this antibody as a direct measure for Mps1 activity at kinetochores (note background centrosomic staining with this antibody is nonspecific and does not change upon Mps1 knockdown or inhibition). As expected, Aurora B inhibition led to a direct reduction in kinetochore-localized Mps1 activity during the early prometaphase ( Fig. 1c ). Figure 1: Aurora B inhibition delays Mps1 activation at kinetochores. ( a ) HeLa cells treated with nocodazole containing DMSO or Hesperadin (100 nM) for 2 h and stained with the indicated antibodies. ( b ) Mean total kinetochore intensities (±s.d.) of Mps1 (dark red bars) or Mad2 (pink bars) relative to centromeres (ACA), treated as in ( a ) or with ZM447439 (2 μM). Data are from 20 cells from two experiments (Hesperadin treatment) or 40 cells from four experiments (DMSO and ZM447439 treatments). Ratios in early prometaphase are set to 1. ( c ) Example immunofluorescent images and quantification of kinetochore signal intensities of Mps1-pT676 over centromeres (ACA) in HeLa cells treated with nocodazole and indicated siRNAs or drugs. ( d ) Example immunofluorescent images and quantification of kinetochore signal intensities of Mad2 over centromeres (ACA) in U2OS cells, non-induced or induced to express LAP–Mis12–Mps1 Δ200 , and treated with nocodazole and indicate drugs. For panels c and d , ratio in si-Mock or DMSO-treated cells is set to 1 and mean data (±s.d.) are from 20 individual cells from two independent experiments. All images most closely resemble the mean values. All standard deviations represent the deviation in mean total kinetochore intensities between all individual cells analysed. Scale bars are 5 μm. For all experiments cells were treated with thymidine for 24 h, released into media containing nocodazole and indicated drugs for 10 h before fixation. siRNAs in panel c were transfected 16 h before the thymidine arrest. Full size image To further ensure that Mad2 loss from kinetochores was a direct consequence of reduced Mps1 activity, we examined whether Mad2 levels could be recovered in Aurora B-inhibited cells when Mps1 activity at kinetochores was restored. We have previously used a Mis12–Mps1 fusion protein to constitutively tether Mps1 to kinetochores [24] . For these purposes, the kinetochore-targeting domain (amino acids 1–200; refs 27 , 29 , AS and GJPLK, unpublished data) was removed to prevent any Aurora B-dependent inputs on Mis12–Mps1. Doxycycline-inducible expression of Mis12–Mps1 Δ200 showed that the fusion protein localized constitutively to kinetochores independently of Aurora B and rescued mitotic checkpoint defects caused by depletion of endogenous Mps1 (GJPLK, unpublished results). Importantly, induced expression of Mis12–Mps1 Δ200 before mitotic entry prevented the reduction in Mad2 kinetochore binding seen following Aurora B inhibition ( Fig. 1d for early prometaphase cells and Supplementary Fig. S2 for all mitotic stages), confirming that the Aurora B-mediated effects on Mad2 are a consequence of impaired Mps1 activity at kinetochores. Furthermore, artificial recruitment of Mps1 to kinetochores before mitosis by inducible expression of Mis12–Mps1 Δ200 caused Mad2 accumulation at kinetochores of G2-phase cells ( Supplementary Fig. S3 ). Although we cannot formally exclude that the rescue by Mis12–Mps1 Δ200 is mediated in part by cytoplasmic functions of Mps1, our observations that high cytoplasmic levels of non-kinetochore-bound Mps1 Δ200 did not rescue Mad2 recruitment or checkpoint activity ( Supplementary Figs S3 and S4 ) strongly suggest that these effects are specifically due to kinetochore-localized Mps1 activity. Collectively, these data demonstrate that Aurora B promotes Mad2 kinetochore binding in early mitosis by localizing Mps1 activity to kinetochores. Aurora B inhibition reduced Mps1 localization to unattached kinetochores throughout mitosis, but it only significantly reduced Mps1 activity at kinetochores during the early stages ( Fig. 1a,b ). Mps1 is thought to auto-activate following local clustering at the kinetochore [8] , [28] , [30] . This may explain why Mps1 activity is merely delayed by Aurora B inhibition, because reducing kinetochore binding would be expected to only delay Mps1 activation. Delays in Mps1 activation can be assessed directly by immunoblotting to observe the hyperphosphorylated state [8] , [25] , [28] if Mps1 activation is synchronously induced. Aurora B inhibition delayed Mps1 hyperphosphorylation in a synchronized Mps1 re-activation assay (see below). Taken together, these data indicate that Aurora B inhibition substantially delays Mps1 activation, but does not altogether prevent it. Rapid Mps1 activation by Aurora B requires Hec1 We hypothesized that Aurora B recruitment to the inner centromere during prophase was responsible for initiating Mps1 recruitment and activation at kinetochores. In strong support of this, artificial recruitment of Aurora B to centromeres before mitosis, by inducible expression of CENPB–INCENP–GFP (CB-INCENP) [31] , caused activation of Aurora B and relocalization of Mps1 to kinetochores of G2-phase cells ( Supplementary Fig. S5 ). To gain more insight into the mechanism by which Aurora B recruits Mps1 to kinetochores, we depleted Ndc80/Hec1 (hereafter referred to as Hec1). Hec1 represented an attractive candidate to mediate kinetochore binding of Mps1 because budding yeast Hec1 directly interacts with Mps1 (ref. 32 ), and is also directly phosphorylated by Aurora B [15] , [16] . Hec1 depletion completely prevented the Aurora B-mediated recruitment of Mps1 to kinetochores in G2 ( Fig. 2a ), inhibited Mps1 recruitment to the kinetochore throughout mitosis and substantially delayed Mps1 activation (as measured by Mad2 recruitment to kinetochores; Fig. 2b,c ). We thus hypothesize that Aurora B–Hec1–Mps1 signal in a linear pathway at the beginning of mitosis to allow Mps1 activation and subsequent Mad2 recruitment to kinetochores. These data agree with earlier findings that Hec1 depletions affect kinetochore binding of Mps1 and imply that the concomitant reduction in Mad2 seen by others [33] , [34] , [35] is due to a delay in Mps1 activation. Mps1 may bind Hec1 directly [32] or, given that Hec1 depletion also affects the localization of many other kinetochore components, may interact with a Hec1-dependent kinetochore protein. 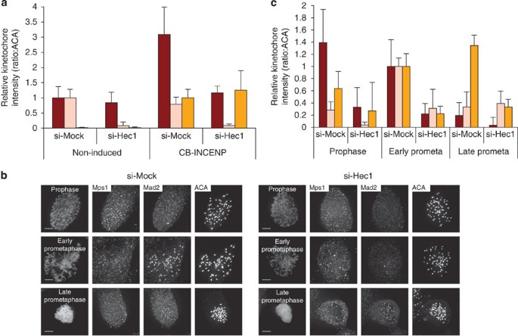Figure 2: Hec1 depletion inhibits Mps1 recruitment and delays activation at kinetochores. (a) Mean total kinetochore intensities (±s.d.) of Mps1 (dark red bars), Hec1 (pink bars) or CB-INCENP (orange bars) relative to centromeres (ACA) in G2-phase U2OS cells (interphase cells 12 h after thymidine release into nocodazole) non-induced or induced to express CB-INCENP (20 cells, two independent experiments). Ratios in si-Mock treatments are set to 1 for non-induced (Mps1 and Hec1) or induced (CB-INCENP) cells. The kinetochore signal for Mps1 seen following si-Hec1 in non-induced controls reflects background staining as it is not reduced by si-Mps1 (results not shown). (b) HeLa cells treated with Mock or Hec1 siRNA and nocodazole before fixation and immunostaining with indicated antibodies. (c) Mean total kinetochore intensities (±s.d.) of Mps1 (dark red bars), Mad2 (pink bars) or Hec1 (orange bars) relative to centromeres (ACA) from 20 cells from two independent experiments, treated as inb. Ratios in early prometaphase si-Mock treatments are set to 1. All images most closely resemble the mean values. All standard deviations represent the deviation in mean total kinetochore intensities between all individual cells analysed. Scale bars are 5 μm. For all experiments cells were transfected with siRNA for 16 h, thymidine added for a further 24 h, before release into media containing nocodazole (−/+ doxycycline in (a)) for 10 h before fixation. Figure 2: Hec1 depletion inhibits Mps1 recruitment and delays activation at kinetochores. ( a ) Mean total kinetochore intensities (±s.d.) of Mps1 (dark red bars), Hec1 (pink bars) or CB-INCENP (orange bars) relative to centromeres (ACA) in G2-phase U2OS cells (interphase cells 12 h after thymidine release into nocodazole) non-induced or induced to express CB-INCENP (20 cells, two independent experiments). Ratios in si-Mock treatments are set to 1 for non-induced (Mps1 and Hec1) or induced (CB-INCENP) cells. The kinetochore signal for Mps1 seen following si-Hec1 in non-induced controls reflects background staining as it is not reduced by si-Mps1 (results not shown). ( b ) HeLa cells treated with Mock or Hec1 siRNA and nocodazole before fixation and immunostaining with indicated antibodies. ( c ) Mean total kinetochore intensities (±s.d.) of Mps1 (dark red bars), Mad2 (pink bars) or Hec1 (orange bars) relative to centromeres (ACA) from 20 cells from two independent experiments, treated as in b . Ratios in early prometaphase si-Mock treatments are set to 1. All images most closely resemble the mean values. All standard deviations represent the deviation in mean total kinetochore intensities between all individual cells analysed. Scale bars are 5 μm. For all experiments cells were transfected with siRNA for 16 h, thymidine added for a further 24 h, before release into media containing nocodazole (−/+ doxycycline in ( a )) for 10 h before fixation. Full size image Checkpoint establishment requires efficient Mps1 activation Initiation of cyclin B degradation in mitosis marks the release of the APC/C from inhibition by the mitotic checkpoint [1] , [36] . To investigate if the delayed Mps1 activation observed upon Aurora B inhibition or Hec1 depletion affected mitotic checkpoint activity, cyclin B–mCherry fluorescence was monitored in real time. Cyclin B levels in nocodazole-treated control cells remained stable for 2 h following nuclear envelope breakdown before slow slippage was initiated (see arrows; Fig. 3a,b ) [37] , indicating potent APC/C inhibition by the mitotic checkpoint. Aurora B inhibition ( Fig. 3a ) or Hec1 depletion ( Fig. 3b ), however, caused rapid degradation of cyclin B as soon as cells entered mitosis. Importantly, cyclin B was subsequently stabilized within 15 min (to a rate approaching that induced by mitotic slippage), indicating that checkpoint establishment was merely delayed ( Fig. 3a,b ). These data imply that checkpoint activation is delayed as a consequence of the delay in Mps1 activation. In support of this, restoring Mps1 activity at kinetochores by the expression of Mis12–Mps1 Δ200 ( Fig. 1d , Supplementary Fig. S2 ) prevented the rapid drop in cyclin B levels following mitotic entry in Aurora B-inhibited or Hec1-depleted cells ( Fig. 3c,d ). The observation that checkpoint establishment is delayed rather than fully inhibited upon addition of Aurora B inhibitors is unlikely to reflect incomplete Aurora B inhibition, because combining Aurora B siRNA with ZM447439 did not further sensitize the checkpoint ( Supplementary Fig. S6 ). 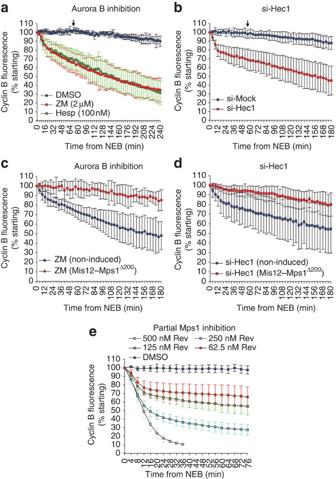Figure 3: Timely establishment of the mitotic checkpoint requires efficient Mps1 activation. Time-lapse imaging of cyclin B–mCherry fluorescence in mitotic U2OS cells treated with nocodazole and (a) indicated inhibitors or (b) siRNA against Hec1. Time-lapse imaging of U2OS cells non-induced or induced to express LAP–Mis12–Mps1Δ200and treated with (c) ZM447439 or (d) Hec1 siRNA. (e) Time-lapse imaging of cyclin B–mCherry fluorescence in mitotic U2OS cells treated with nocodazole and indicated concentrations of reversine. Arrows ina,bindicate start of mitotic slippage. Fluorescence at nuclear envelope breakdown (NEB) was set to 100%. Data represent the mean (±s.d.) of at least 6–10 cells, which is representative of at least three independent experiments. All drugs were added before mitotic entry. For all siRNA experiments cells were transfected for 16 h, thymidine added for a further 24 h, and cells released into media containing nocodazole (−/+ doxycycline in (d)). Figure 3: Timely establishment of the mitotic checkpoint requires efficient Mps1 activation. Time-lapse imaging of cyclin B–mCherry fluorescence in mitotic U2OS cells treated with nocodazole and ( a ) indicated inhibitors or ( b ) siRNA against Hec1. Time-lapse imaging of U2OS cells non-induced or induced to express LAP–Mis12–Mps1 Δ200 and treated with ( c ) ZM447439 or ( d ) Hec1 siRNA. ( e ) Time-lapse imaging of cyclin B–mCherry fluorescence in mitotic U2OS cells treated with nocodazole and indicated concentrations of reversine. Arrows in a , b indicate start of mitotic slippage. Fluorescence at nuclear envelope breakdown (NEB) was set to 100%. Data represent the mean (±s.d.) of at least 6–10 cells, which is representative of at least three independent experiments. All drugs were added before mitotic entry. For all siRNA experiments cells were transfected for 16 h, thymidine added for a further 24 h, and cells released into media containing nocodazole (−/+ doxycycline in ( d )). Full size image If Aurora B inhibition affects checkpoint establishment by decreasing the efficiency of Mps1 activation at the kinetochore, partial Mps1 inhibition may cause similar delays in checkpoint establishment. Suboptimal doses (≤500 nM) of the Mps1 inhibitor reversine [25] caused inefficient Mps1 activation (as measured by delayed Mad2 kinetochore binding) and faster mitotic exit ( Supplementary Figs S7 and S8a ). Strikingly, increasing concentrations of reversine (62–500 nM) caused increasing delays in checkpoint establishment, as measured by Cyclin B stabilization in nocodazole ( Fig. 3e ). Aurora B synergises with Hec1 and Mps1 Although potent Mps1 inhibition and penetrant Hec1 depletion abrogate mitotic checkpoint activity [8] , [9] , [10] , [25] , [27] , [35] , potent Aurora B inhibition does not. We hypothesized that if Aurora B and Hec1 are important for Mps1 to initiate checkpoint signalling, the checkpoint might be sensitized to Aurora B inhibition when downstream components of the pathway are functionally compromised. Indeed, inhibition or knockdown of any two individual components was functionally synergistic against the mitotic checkpoint response to nocodazole, as judged by measuring the cumulative frequency of cells that exited mitosis at defined times after nuclear envelope breakdown ( Fig. 4a–c ). For instance, although a low dose of reversine (125 nM) or 2 μM ZM447439 alone allowed cells to arrest in nocodazole for many hours, combining both compounds caused exit within 30 min ( Fig. 4a ). Given that potent Mps1 inhibition achieved similar fast exit (see Supplementary Fig. S8a,b ), this is likely to reflect complete inactivation of the mitotic checkpoint. The synergy between Aurora B and partial Mps1 inhibition occurred over a range of reversine doses ( Supplementary Fig. S8a ), and was further confirmed with an independent Mps1 inhibitor, Mps1-IN-1 ( Supplementary Fig. S8b ) [9] , as well as with siRNA-mediated depletion of Mps1 and Aurora B ( Supplementary Figs S6 and S8c ). Furthermore, using a high dose of nocodazole (3.2 μM, see ref. 13 ) showed that this effect of Aurora B inhibition was not due to possible effects of Aurora B on residual microtubules ( Supplementary Fig. S8d,e ). 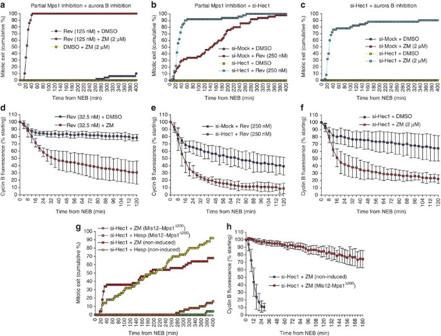Figure 4: Aurora B, Hec1 and Mps1 synergize to establish the mitotic checkpoint. (a–c) Time-lapse analysis of duration of mitotic arrest in HeLa cells treated with nocodazole after combinations of siRNA and/or inhibitors, as indicated. Data indicate cumulative percentage of cells (from 50 cells per treatment) that exit mitosis (scored as cell flattening) at the indicated times after NEB, and are representative of 2–5 independent experiments. (d–f) Cyclin B–mCherry fluorescence of U2OS cells treated with nocodazole in combination of siRNA and/or inhibitors, as indicated. In d, 32.5 nM reversine was used to observe the long mitotic delay, as this prevented fast mitotic exit in all cells following ZM447439 addition. Ineandf, means for si-Hec + inhibitors were calculated from cells that did not exit mitosis within 2 h. (g) Time-lapse analysis of duration of mitotic arrest in U2OS cells treated with Hec1 siRNA and indicated inhibitors in cells non-induced or induced to express LAP–Mis12–Mps1Δ200. Data indicate cumulative percentage of cells (from 50 cells per treatment) that exit mitosis (scored as cell flattening) at the indicated times after NEB, and are representative of three independent experiments.(h) Cyclin B–mCherry fluorescence of U2OS cells treated with Hec1 siRNA and ZM447439 and non-induced or induced to express LAP–Mis12–Mps1Δ200. Data fromd,e,fand h are means (±s.d.) of 6–8 individual cells, which is representative of 2–3 independent experiments. Fluorescence at nuclear envelope breakdown (NEB) ind,e,fandhwas set to 100%. All drugs were added before mitotic entry. Figure 4: Aurora B, Hec1 and Mps1 synergize to establish the mitotic checkpoint. ( a–c ) Time-lapse analysis of duration of mitotic arrest in HeLa cells treated with nocodazole after combinations of siRNA and/or inhibitors, as indicated. Data indicate cumulative percentage of cells (from 50 cells per treatment) that exit mitosis (scored as cell flattening) at the indicated times after NEB, and are representative of 2–5 independent experiments. ( d – f ) Cyclin B–mCherry fluorescence of U2OS cells treated with nocodazole in combination of siRNA and/or inhibitors, as indicated. In d, 32.5 nM reversine was used to observe the long mitotic delay, as this prevented fast mitotic exit in all cells following ZM447439 addition. In e and f , means for si-Hec + inhibitors were calculated from cells that did not exit mitosis within 2 h. ( g ) Time-lapse analysis of duration of mitotic arrest in U2OS cells treated with Hec1 siRNA and indicated inhibitors in cells non-induced or induced to express LAP–Mis12–Mps1 Δ200 . Data indicate cumulative percentage of cells (from 50 cells per treatment) that exit mitosis (scored as cell flattening) at the indicated times after NEB, and are representative of three independent experiments. (h ) Cyclin B–mCherry fluorescence of U2OS cells treated with Hec1 siRNA and ZM447439 and non-induced or induced to express LAP–Mis12–Mps1 Δ200 . Data from d , e , f and h are means (±s.d.) of 6–8 individual cells, which is representative of 2–3 independent experiments. Fluorescence at nuclear envelope breakdown (NEB) in d , e , f and h was set to 100%. All drugs were added before mitotic entry. Full size image In line with the fact that Aurora B inhibition or partial Mps1 inhibition only delayed establishment of the checkpoint ( Fig. 3 ), combining Aurora B inhibitor with a very low dose of reversine (32.5 nM) resulted in a significantly longer delay, as measured by cyclin B fluorescence ( Fig. 4d ). Strikingly, the few cells that did not rapidly exit mitosis when treated with Hec1 siRNA combined with either a higher dose of reversine (250 nM) or Aurora B inhibitor (see Fig. 4b,c ) had degraded cyclin B almost completely before checkpoint signalling was capable of stabilizing it ( Fig. 4e,f ). The fast mitotic exit in nocodazole induced by Hec1 depletion combined with ZM447439 or Hesperadin treatment was prevented by Mis12–Mps1 Δ200 expression ( Fig. 4g ). Moreover, induction of Mis12–Mps1 Δ200 also completely prevented any drop in cyclin B levels upon mitotic entry, indicating that the checkpoint was still initiated maximally as soon as cells enter mitosis if Mps1 was preserved at kinetochores ( Fig. 4h ). These data demonstrate that the synergy between Aurora B inhibition and Hec1 depletion, also shown recently by others [38] , prevents mitotic checkpoint signalling because it causes long delays in Mps1 activation and checkpoint establishment. In the majority of cells, the delay is long enough to prevent checkpoint activation before cyclin B degradation is complete and mitotic exit is initiated. Furthermore, the recruitment of Mps1 to kinetochores is the primary role for Aurora B and Hec1 in mitotic checkpoint signalling, because recovering Mps1 activity at kinetochores bypasses all checkpoint phenotypes associated with Aurora B inhibition and/or Hec1 depletion. Aurora B is not critical to maintain Mps1 activity Our data support the hypothesis that Aurora B co-operates with Hec1 to allow efficient Mps1 activation and checkpoint establishment at the beginning of mitosis. Hec1 depletion sensitized the checkpoint to Aurora B inhibition ( Fig. 4c ); however, we observed no additional sensitization when combining Aurora B inhibitors with Aurora B siRNAs ( Supplementary Fig. S6 ). Therefore, we predict that Aurora B is an amplifier rather than an essential component required for Mps1 activation at kinetochores. This amplifier allows rapid checkpoint establishment at mitotic onset, but is less important thereafter (at least in the continued presence of nocodazole; Fig. 3a ). To address whether Aurora B was required at all to maintain the checkpoint after Mps1 activation is achieved, cyclin B levels were monitored in nocodazole-treated cells that received Aurora B inhibitor after mitotic entry. 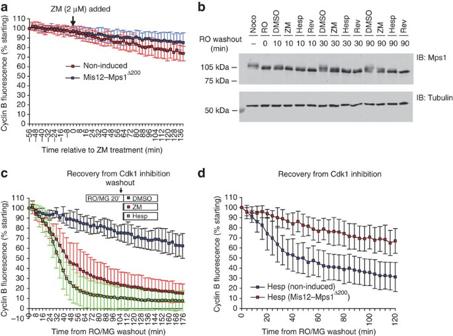Figure 5: Aurora B is primarily needed to establish Mps1 activity. (a) Time-lapse imaging of cyclin B–mCherry fluorescence in mitotic U2OS cells either non-induced or induced to express Mis12–Mps1Δ200and treated with nocodazole before addition of ZM447439. The time is plotted relative to ZM addition (which is indicated by an arrow). The cyclin B intensity of the first image, which is 15 frames before ZM addition, was set to 100%. The mean data (±s.d.) is plotted from eight cells, which is representative of two independent experiments. (b) Immunoblot of whole cell lysates from HeLa cells treated with nocodazole without (−) or with 20 min RO3306 treatment (all other lanes) and subsequently released into nocodazole/inhibitor for the indicated times. (c) Time-lapse imaging of cyclin B–mCherry fluorescence in mitotic U2OS cells treated with nocodazole for 2 h, including RO3306/MG132 (RO/MG) for the final 20 min. Cells were subsequently released into nocodazole plus the indicated inhibitors. Please note that Cdk1 inhibition in noco/MG132-treated cells for only 20 min did not cause mitotic exit as we observed no visible chromosome decondensation39. (d) Time-lapse imaging of cyclin B–mCherry fluorescence, performed exactly as in c, in U2OS cells non-induced or induced to express LAP–Mis12–Mps1Δ200before mitotic entry. The mean data (±s.d.) in c and d are plotted from 6–8 cells, which is representative of three independent experiments. As shown in Figure 5a , ZM447439 addition caused a slight weakening of the checkpoint when given to cells already arrested in nocodazole. This moderate effect was prevented by expression of Mis12–Mps1 Δ200 ( Fig. 5a ), showing that Aurora B still impacted to some extent the ability of Mps1 to maintain the checkpoint during mitosis. Interestingly, Mps1 autophosphorylation sites that are required for its activity [28] , [30] displayed slow turnover, as inhibiting Mps1 kinase activity during mitosis with 1 μM reversine was unable to cause dephosphorylation of Mps1 (pT676 and mobility shift; Supplementary Fig. S9 ). In contrast, mitotic exit (lane 6 of Supplementary Fig. S9 ) or cdk1 inhibition (lane 3 of Supplementary Fig. S9 ) efficiently dephosphorylated and thus inactivated Mps1. This suggests that once activated, Mps1 no longer relies on activating inputs to be maintained in its active, hyperphosphorylated state during mitosis, possibly explaining the limited effect of Aurora B inhibition on the checkpoint when applied during a nocodazole arrest. To test this, we returned Mps1 to its hypophosphorylated, inactive state by inhibition of cdk1 and asked whether it could re-activate in mitosis in the absence of Aurora B activity. Nocodazole-arrested cells were treated with the cdk1 inhibitor RO3306 (combined with MG132 to prevent cyclin B degradation), which caused rapid dephosphorylation of Mps1 within 20 min ( Fig. 5b , Supplementary Fig. S9 ). Treatment was limited to 20 min to prevent mitotic exit (all chromosomes remained visibly condensed) [39] . Although release from RO3306/MG132 quickly re-established Mps1 activity as well as mitotic checkpoint function, both were severely delayed when cells were released from cdk1 inhibition in the presence of Aurora B inhibitors ( Fig. 5b,c ). This dependence on Aurora B was not observed if recovery from cdk1 inhibition was performed in cells induced to express Mis12–Mps1 Δ200 ( Fig. 5d ). Figure 5: Aurora B is primarily needed to establish Mps1 activity. ( a ) Time-lapse imaging of cyclin B–mCherry fluorescence in mitotic U2OS cells either non-induced or induced to express Mis12–Mps1 Δ200 and treated with nocodazole before addition of ZM447439. The time is plotted relative to ZM addition (which is indicated by an arrow). The cyclin B intensity of the first image, which is 15 frames before ZM addition, was set to 100%. The mean data (±s.d.) is plotted from eight cells, which is representative of two independent experiments. ( b ) Immunoblot of whole cell lysates from HeLa cells treated with nocodazole without (−) or with 20 min RO3306 treatment (all other lanes) and subsequently released into nocodazole/inhibitor for the indicated times. ( c ) Time-lapse imaging of cyclin B–mCherry fluorescence in mitotic U2OS cells treated with nocodazole for 2 h, including RO3306/MG132 (RO/MG) for the final 20 min. Cells were subsequently released into nocodazole plus the indicated inhibitors. Please note that Cdk1 inhibition in noco/MG132-treated cells for only 20 min did not cause mitotic exit as we observed no visible chromosome decondensation [39] . ( d ) Time-lapse imaging of cyclin B–mCherry fluorescence, performed exactly as in c, in U2OS cells non-induced or induced to express LAP–Mis12–Mps1 Δ200 before mitotic entry. The mean data (±s.d.) in c and d are plotted from 6–8 cells, which is representative of three independent experiments. Full size image These data demonstrate that Aurora B works together with Hec1 (or a Hec1-dependent kinetochore protein) to recruit Mps1 to kinetochores during mitosis. This pathway is essential to rapidly activate Mps1 at the onset of mitosis and thus ensure the checkpoint is efficiently engaged. A critical role for Aurora B in mounting a checkpoint response to unattached kinetochores has not previously been shown in mammalian cells, largely due to the fact that potent Aurora B inhibitors have been ineffective at preventing a nocodazole-induced mitotic delay [13] , [22] , [23] . Some studies, however, reported that such delays are significantly less pronounced when Aurora B is inhibited [22] , [23] . Our data explain why Aurora B inhibitors are ineffective in nocodazole-treated cells and why these cells nevertheless exit faster than control cells. We propose that establishment of the checkpoint is merely delayed when Aurora B is inhibited, which is a direct result of a delay in Mps1 activation. When the checkpoint is eventually established, cells proceed with reduced cyclin B levels and slippage subsequently steadily reduces the remaining cyclin B (at a slightly accelerated rate) until cells eventually exit mitosis after several hours. Therefore Aurora B inhibitors are effective at overriding the checkpoint in nocodazole, but primarily during the very early stages of mitosis. Interestingly, a recent study showed both Aurora B and Mps1 were required to propagate a mitotic checkpoint response on fully bioriented chromosomes when Mad1 was constitutively tethered to kinetochores [40] . It will be interesting to examine whether, under these conditions, Mps1 activity also relies on Aurora B-dependent recruitment to kinetochores. Why then does Aurora B activity cease being critical to maintain a checkpoint when Mps1 activity has been established? Our data indicate that Aurora B merely amplifies Mps1 recruitment to kinetochores, which is important upon mitotic entry when Mps1 must auto-activate efficiently to ensure that the mitotic checkpoint is engaged on time. Following this initial activation, however, the requirements for Aurora B may be relaxed while all kinetochores are able to functionally recruit active Mps1 and thereby propagate the checkpoint. However, this may only be a temporary reprieve, because as chromosomes congress the checkpoint would need to be maintained with progressively fewer unattached kinetochores. Although technically challenging, it will be important to address whether the checkpoint is more sensitive to Aurora B inhibitors in cells containing only few unattached kinetochores. Hec1 is likely to be essential for Mps1 localization at kinetochores, given that Hec1 depletion combined with Aurora B inhibition is very effective at overriding the checkpoint in nocodazole and yet this is still completely prevented by recovering Mps1 at kinetochores. This would explain the complete checkpoint override following efficient Hec1 depletion seen by others [35] , although it remains to be formally tested whether recovering Mps1 recruitment would similarly recover the checkpoint response under these conditions. Ultimately, it will be critical to address whether Mps1 binds directly to Hec1 and, if so, how Aurora B-mediated phosphorylation(s) impacts on this association. A likely hypothesis, based on our data and the direct biochemical interaction between the Hec1 N terminus and Mps1 in budding yeast [32] , is that Aurora B-mediated phosphorylation of the Hec1 N-terminal tail potentiates direct interaction with Mps1. Finally, we have previously shown that Mps1 enhances activation of Aurora B [41] , and that this is most apparent when cells enter mitosis with reduced Mps1 activity [10] . This suggests the possibility that Mps1 and Aurora B are engaged in a positive feedback loop that ensures rapid establishment of both the mitotic checkpoint and error-correction pathways at the beginning of mitosis. Experiments are underway to test this hypothesis. Cell culture and reagents HeLa cells were grown in DMEM supplemented with 8% fetal bovine serum, penicillin/streptomycin and L -glutamine (2 mM). All doxycycline-inducible cells lines were derived from U2OS-TR (a gift from M. Timmers) cultured in the same media but containing 8% Tet-approved fetal bovine serum (Clontech), and protein expression was induced by doxycycline addition (at 1 μg ml −1 ) for at least 6 h. Thymidine (2.5 mM), nocodazole (830 nM), taxol (1 μM), MG132 (5 μM), reversine (various doses), doxycycline, G-418 (1 mg ml −1 ) and puromycin (1 μg ml −1 ) were all from Sigma. Zeocin (100 μg ml −1 ) was from Invitrogen. RO3306 (Enzo Life Sciences) was used at 10 μM, ZM447449 (Tocris Bioscience) at 2 μM, Hesperadin (Selleck Chemicals) at 100 nM and Mps1-IN-1 (gift from Nathanael Gray) at 10 μM throughout, unless stated otherwise. Cell lines The U2OS-TR cell line was transfected with pcDNA4 vector (Invitrogen) encoding LAP–Mis12–Mps1 Δ200 , LAP–Mps1 Δ200 or CB-INCENP–GFP and selected with Zeocin. Monoclonal cells lines were then established by limited dilution (Clone 9B; LAP–Mis12–Mps1 Δ200 , Clone 23; LAP–Mps1 Δ200 , Clone 6 CB-INCENP–GFP). Stable lines coexpressing cyclin B–mCherry were subsequently created by transfection of cyclin B–mCherry (based on a pEGP-N1 vector backbone; kind gift from R. Wolthuis) and selection with G-418. An inducible cyclin B U2OS-TR clone (Clone 3) was obtained by co-transfecting pcDNA5 encoding cyclin B–mCherry with pBabe-puro (10:1 ratio), selecting with puromycin and single cell cloning. Antibodies The following primary antibodies were used for immunofluorescence imaging and immunoblotting (at indicated final concentrations): Mps1-NT (Upstate; 0.5 μg ml −1 ), pT676-Mps1 [28] (1 μg ml −1 ), Mad2 (ref. 10 ; 0.5 μg ml −1 ), α-tubulin (Sigma; 0.2 μg ml −1 ), CREST/ACA (Fitzgerald Industry Int; 0.5 μg ml −1 ), Aurora B (AIM, BD transduction; 0.25 μg ml −1 ), pT232-Aurora B (Rockland; 0.5 μg ml −1 ), Hec1 (9G3, Abcam; 1 μg ml −1 ), cyclin B (H-433, Santa Cruz; 0.2 μg ml −1 ). Secondary antibodies were high-crossed absorbed goat-anti-human Alexafluor647, goat-anti-rabbit and anti-mouse Alexafluor488 and Alexafluor568 (Molecular Probes) for immunofluorescence studies, and anti-Mouse/Rabbit-HRP (Bio-Rad) for immunoblotting. Plasmids and siRNAs LAP–Mis12–Mps1, LAP–Mps1 and CB-INCENP–GFP have been described [24] , [31] , [41] , [42] . LAP–Mis12–Mps1 Δ200 or LAP–Mps1 Δ200 were constructed using Quickchange mutagenesis to create a Xho1 site at 600 bp, which was used to excise the first 600 bases of Mps1 from either LAP–Mis12–Mps1 or LAP–Mps1. Plasmids were transfected using Fugene 6 (Roche) according to the manufacturer's instructions. siRNAs used in this study were as follows: si-Hec1 (5′-AAGU UCAAAAGCUGGAUGAUC-3′, custom; Dharmacon), si-Mps1 (5′-GACAGAU GAUUCAGUUGUA-3′, custom; Dharmacon), si-Mock (Luciferase GL2 duplex; Dharmacon/D-001100-01-20) and si-AurB (ON-TARGETplus si-RNA J-003326-23, AURBKB, Dharmacon). All siRNAs were transfected using Hiperfect (Qiagen) at 20 nM according to the manufacturer's instructions. Live cell imaging and immunfluorescence For live cell imaging, cells were plated in four-well or eight-well chambered glass-bottom slides (LabTekII) or 24-well glass-bottom plates (MatTek), transfected and imaged in a heated chamber (37°C and 5% CO 2 ) using a ×10/0.3NA CPlanFLN or ×20/0.5NA UPLFLN objective on a Olympus IX-81 microscope, controlled by Cell-M software (Olympus). Images were acquired using a Hamamatsu ORCA-ER camera and processed using Cell-M software. For immunofluorescence studies, cells plated on 12-mm coverslips, were pre-extracted with 0.2% Triton X-100 in PEM (100 mM PIPES (pH 6.8), 1 mM MgCl 2 and 5 mM EGTA) for 45 s before fixation with 4% paraformaldehyde in PBS (for Mps1, Mad2 and Hec1). Aurora B and pAurB stainings were performed on cells fixed directly in 4% paraformaldehyde. Coverslips were blocked with 2% bovine serum albumin in PBS/0.1% Triton for 15 min, incubated with primary antibody for 16 h at 4 °C, washed with PBS, and incubated with secondary antibodies and 4,6-diamidino-2-phenylindole for an additional 2 h at room temperature. Coverslips were washed and mounted using ProLong antifade (Molecular Probes). All images were acquired on a DeltaVision RT system (Applied Precision) with a ×100/1.40NA UPlanSApo objective (Olympus) using SoftWorx software. Images are maximum intensity projections of deconvolved stacks. For quantification of immunostaining, all images of similarly stained experiments were acquired with identical illumination settings and analysed using ImageJ. An ImageJ macro was designed to threshold and select all centromeres and all chromosomes areas (excluding centromeres), using the 4,6-diamidino-2-phenylindole and ACA channels. The convolve filter was first applied to the ACA channel and the threshold selection increased by 1 pixel (to ensure complete kinetochore selection). This was used to calculate the relative mean kinetochore intensity of Mad2, Mps1 and Hec1 ([centromere–chromosome arm intensity (Mad2/Mps1/Hec1)]/[centromere–chromosome arm intensity (ACA)]). For centromere localization of AurB/pAurB, a true background outside the cell was used to subtract from the centromere intensity (and centromere areas were enlarged by 3 pixels to incorporate the more diffuse Aurora B staining). For quantification of cyclin B–mCherry fluorescence, ImageJ was used to calculate the total integrated fluorescence intensity of individual cells at each time point (after background subtraction of all images using a rolling ball radius of 200 pixels). For all kinetochore intensity quantifications, means and standard deviations were calculated for each individual experiment and then combined using the standard method for non-overlapping data sets. How to cite this article: Saurin, A. T. et al . Aurora B potentiates Mps1 activation to ensure rapid checkpoint establishment at the onset of mitosis. Nat. Commun. 2:316 doi: 10.1038/ncomms1319 (2011).